Structural signatures of dynamic heterogeneities in monolayers of colloidal ellipsoids When a liquid is supercooled towards the glass transition, its dynamics drastically slows down, whereas its static structure remains relatively unchanged. Finding a structural signature of the dynamic slowing down is a major challenge, yet it is often too subtle to be uncovered. Here we discover the structural signatures for both translational and rotational dynamics in monolayers of colloidal ellipsoids by video microscopy experiments and computer simulations. The correlation lengths of the dynamic slowest-moving clusters, the static glassy clusters, the static local structural entropy and the dynamic heterogeneity follow the same power-law divergence, suggesting that the kinetic slowing down is caused by a decrease in the structural entropy and an increase in the size of the glassy cluster. Ellipsoids with different aspect ratios exhibit single- or double-step glass transitions with distinct dynamic heterogeneities. These findings demonstrate that the particle shape anisotropy has important effects on the structure and dynamics of the glass. The nature of the glass transition is one of the major unsolved mysteries in physics [1] , [2] , [3] . On approaching the glass transition, the dynamics becomes not only progressively slower but also more spatially heterogeneous [1] , [2] . Whether such dynamic heterogeneity (DH) is associated with any structural change is a central problem and an important theoretical assumption in glass transition studies [2] , [4] , [5] , [6] , [7] , [8] . Two types of structure signatures, amorphous order [2] , [4] , [6] , [9] and crystalline order [8] , have been proposed as responsible for the dynamics arrest. As an archetypal model of amorphous order, icosahedral order was often considered to be crucial for vitrification in systems of spheres [9] , [10] , [11] , and its percolation was associated with the glass transition [12] . On the other hand, the ground-state crystalline structure, even if avoided, is suggested to be important for the glass transition [8] . Recently, crystalline clusters with low structural entropy were shown to be responsible for the dynamic arrest in systems of spheres [13] , [14] , [15] . Despite the intensive search for the structural origin of slow dynamics in glass transitions, little is known for systems of anisotropic particles. Here we employ colloidal ellipsoids that rarely exhibit local crystalline order or icosahedral order studied in systems of spheres. By identifying the static glassy particles and determining the local structural entropies for anisotropic particles, we discover novel structural signatures of DHs in both experiments and simulations, and confirmed that the glassy clusters with low structural entropy are responsible for dynamic arrest not only in translational degrees of freedom [13] , [14] , [15] , but also in rotational degrees of freedom. Colloids are considered as outstanding model systems for glass transition studies because trajectories of individual particles can be directly measured by video microscopy [16] , [17] , [18] . Significant insights into the glass transition have been obtained from experiments on colloidal spheres [17] , [18] , [19] , [20] . Anisotropic particles, by contrast, are much less frequently used as a model system in such studies [21] , [22] , [23] , [24] , despite the fact that they can better mimic molecules with anisotropic shapes or interactions. Monodisperse ellipsoids are excellent glass formers in two dimensions (2D) because their shape can effectively frustrate crystallization and quasi-long-range nematic order [22] , [25] . Here we study the glass transitions in monolayers of colloidal ellipsoids. The quasi-2D sample enables us to better image and track particle motion. The anisotropic shape of the particles makes both translational and rotational motion measurable. We used four batches of polymethyl methacrylate (PMMA) ellipsoids with aspect ratios P = a/b =2.3, 3.5, 6.0 and 9.0, where a and b are the semi-major and semi-minor axes, respectively. All the ellipsoids were obtained by stretching spheres with a diameter of 2.0 μm. A monolayer of ellipsoids was dispersed in water between two parallel horizontal glass walls. For colloids in 2D, the area fraction ϕ ≡ πabρ plays a similar role as the inverse temperature 1/ T in molecular systems [16] , [17] . Here ρ is the number density. About 10 area fractions within 0.20≤ ϕ ≤0.86 were studied for each aspect ratio by video microscopy. During the 3- to 6-h measurements at each ϕ , no drift flow or density change was observed. The Brownian motion of ~6,000 ellipsoids in the field of view was typically recorded at one frame per second. The center-of-mass positions and orientations of individual ellipsoids were tracked using our image-processing algorithm [26] . In this paper, we focus on the development of DH, the evolution of static structures and their relationships towards the glass transition at different aspect ratios. First, we characterize the kinetic phase behaviour at different aspect ratios by measuring the mode-coupling critical point ϕ c and the ideal glass transition point ϕ 0 from the fits to the structural relaxation times as a function of density [3] , [22] , [27] . Next, we measure the DHs by directly visualizing the spatial distribution of fast translational (FT), fast rotational (FR), slow translational (ST) and slow rotational (SR) particles and by measuring the four-point dynamic correlations [2] , [28] . Finally, we analyse the static structures by identifying glassy particles and measuring local structural entropy. From these analyses in both translational and rotational degrees of freedom, we find the following structural signatures of the dynamic slowing down in monolayers of ellipsoids: the static glassy (that is, high number of neighbours for translational motion and high nematic order for orientational motion) clusters correspond to low structural entropy and are highly correlated to clusters with the slowest dynamics, thereby suggesting that the kinetic slowing down is caused by a decrease in the structural entropy and a increase in the size of the glassy clusters. This indicates that it is the growth of glassy clusters with low structural entropy that dictates the dynamic arrest rather than the local crystalline order or particular amorphous order, which rarely exists in systems of ellipsoids. Phase behaviour The equilibrium and non-equilibrium phase behaviour of ellipsoids in 2D can be qualitatively described as follows ( Fig. 1 ). When the aspect ratio P =1, monodisperse disks only form crystals or polycrystals even under the fastest quench to high density in experiment and simulation. For P ≃ 1, ellipsoids resemble circular disks and form 2D crystals with free rotational motion owing to the spacing between them ( Fig. 1b ). This rotator phase or plastic crystal in 2D has quasi-long-range translational order and short-range nematic orientational order. As P → ∞ , ellipsoids would form a nematic phase ( Fig. 1e ) with quasi-long-range orientational order and short-range translational order [29] . Ellipsoids with intermediate P tend to form local splay structures at high density ( Fig. 1f ), so that the system has neither quasi-long-range translational order nor quasi-long-range orientational order, that is, a glass. Moreover, glasses with pseudonematic domains may form at large P ( Fig. 1d ), and glasses without domains may form at small P ( Fig. 1c ). The molecular mode-coupling theory [30] predicts similar glasses for ellipsoids in three dimensions, including an orientational glass at P ≳ 2.5 where rotational motion becomes glassy while the translational motion remains quasi-ergodic [31] . Simulations about glass of ellipsoids mainly focused on small aspect ratios in 2D [25] , [32] , [33] . The recent simulation about ellipses in 2D indicates that the rotational glass transition should be at a lower density than the translational one for P >3, while at a higher density for P <2 (ref. 34 ). The orientational glass has been observed experimentally in quasi-2D systems of colloidal ellipsoids with P= 6 (ref. 22 ). Here we found that the 2D orientational glass region shrinks as P decreases and completely vanishes at P ≃ 2.5. 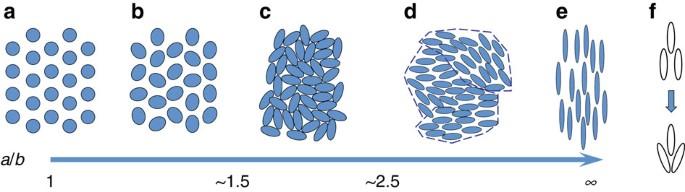Figure 1: Equilibrium and non-equilibrium phases of hard ellipses in 2D. As the aspect ratioP=a/bincreases, ellipses form (a) a crystal, (b) a rotator phase, (c) a conventional glass without pseudonematic domains, (d) an orientational glass with pseudonematic domains and (e) a nematic phase. (f) Three closely packed ellipses tend to have slightly different orientations. Figure 1: Equilibrium and non-equilibrium phases of hard ellipses in 2D. As the aspect ratio P = a / b increases, ellipses form ( a ) a crystal, ( b ) a rotator phase, ( c ) a conventional glass without pseudonematic domains, ( d ) an orientational glass with pseudonematic domains and ( e ) a nematic phase. ( f ) Three closely packed ellipses tend to have slightly different orientations. Full size image We quantitatively measure the glass transition densities from the translational and rotational relaxations characterized by the self-intermediate scattering function and the orientational correlation function , respectively [25] . x j ( t ) and θ j ( t ) are the position and orientation of ellipsoid j at time t , q is the scattering vector, n is a positive integer, N is the total number of particles and ‹ › denotes the ensemble average. We chose q = q m corresponding to the first peak in the structure factor at high density and n =3 in Fig. 2 . Different choices of q and n yield the same glass transition points ( Fig. 3c,f ). At high ϕ , both F s ( t ) and L n ( t ) develop a two-step relaxation, a signature of glassy dynamics. According to the mode-coupling theory, the long-time α-relaxation follows the Kohlrausch law e − ( t / τ ) β (ref. 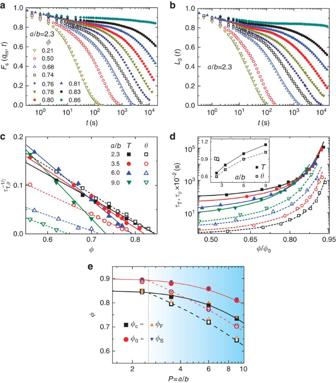Figure 2: Single-step and double-step glass transitions at different aspect ratios. (a)Fs(qm,t) and (b)L3(t) for ellipsoids with aspect ratioP=a/b=2.3. (c) The translational relaxation time τT(solid symbols) and rotational relaxation time τθ(open symbols) fitted with equation (1). (d) τT(solid symbols) and τθ(open symbols) fitted with equation (2). Inset: the fitted fragility indexB. (e) The measuredϕc(equation (1)),ϕ0(equation (2)),ϕF(equation (3)) andϕS(equation (4)) for translational (solid symbols) and rotational (open symbols) motion all show a single-step glass transition atP≲2.5 and a double-step transition atP≳2.5. Curves are guides to the eye. 27 ) and the structural relaxation time τ follows Figure 2: Single-step and double-step glass transitions at different aspect ratios. ( a ) F s ( q m , t ) and ( b ) L 3 ( t ) for ellipsoids with aspect ratio P = a / b =2.3. ( c ) The translational relaxation time τ T (solid symbols) and rotational relaxation time τ θ (open symbols) fitted with equation (1). ( d ) τ T (solid symbols) and τ θ (open symbols) fitted with equation (2). Inset: the fitted fragility index B . ( e ) The measured ϕ c (equation (1)), ϕ 0 (equation (2)), ϕ F (equation (3)) and ϕ S (equation (4)) for translational (solid symbols) and rotational (open symbols) motion all show a single-step glass transition at P ≲ 2.5 and a double-step transition at P ≳ 2.5. Curves are guides to the eye. 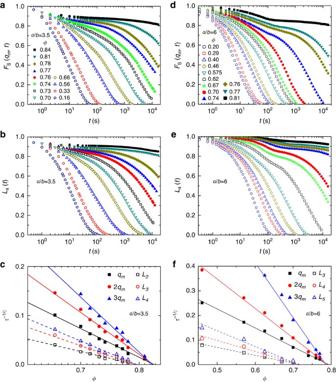Figure 3: Translational and rotational relaxations. (a–c)P=3.5; (d–f)P=6.0. (a)Fs(qm,t) atqm=1.9 μm−1. (d)Fs(qm,t) atqm=2.3 μm−1. (b,e)L4(t). Legends in (b,e) are the same as those in (a,d), respectively. (c,f) The translational relaxation time τT(solid symbols) and rotational relaxation time τθ(open symbols) fitted with equation (1) (solid and dashed straight lines). Full size image Figure 3: Translational and rotational relaxations. ( a – c ) P =3.5; ( d – f ) P =6.0. ( a ) F s ( q m , t ) at q m =1.9 μm −1 . ( d ) F s ( q m , t ) at q m =2.3 μm −1 . ( b , e ) L 4 ( t ). Legends in ( b , e ) are the same as those in ( a , d ), respectively. ( c , f ) The translational relaxation time τ T (solid symbols) and rotational relaxation time τ θ (open symbols) fitted with equation (1) (solid and dashed straight lines). Full size image where ϕ c is the critical glass transition point, and γ is obtained from fitting the α- and β-relaxations [27] . Translational τ T and rotational τ θ obtained from Fig. 2a,b can both be well fitted with equation (1); ( Fig. 2c ). The fitted for P =2.3 indicates a single-step glass transition (supercooled liquid→glass), while for P =3.5, 6.0 and 9.0 ( Figs 2c and 3c,f ) corresponds to a double-step glass transition (supercooled liquid→orientational glass→glass). This agrees with the observation that ellipsoids form pseudonematic domains only at P ≳ 2.5 such that they no longer rotate but still glide translationally within the domains, a signature of an orientational glass [22] , [31] . Figure 2d shows that the relaxation time is also satisfactorily fitted with the Vogel–Fulcher–Tammann equation where ϕ 0 is the ideal glass transition point and B is the fragility index [3] , [4] . Both the fitted ϕ 0 and ϕ c shown in Fig. 2e confirm the single-step glass transition at P ≲ 2.5 and the double-step glass transition at P ≳ 2.5. ϕ 0 > ϕ c because all structural relaxations cease at ϕ 0, while only free-diffusion relaxations become kinetically arrested at ϕ c (refs 1 , 3 ). A smaller B represents a more fragile liquid whose viscosity or τ is more sensitive to a change in T or ϕ . Fragility is the key concept in the search for a universal description of dynamic arrest in glass-forming liquids, but its physical origin is still lacking. Recent experiments by Mattsson et al. [19] have shown that softer colloidal spheres lead to a stronger (less fragile) glass. Here we observed that a larger aspect ratio similarly gives a less-fragile glass (inset of Fig. 2d ). This behaviour was observed in recent simulations on rods [35] , but has not been tested in experiment before. We performed kinetic Monte Carlo (kMC) simulations to mimic the Brownian motion of 5,000 ellipses. The same structural relaxations, glass transitions and fragility behaviours were reproduced as shown in Fig. 4 . 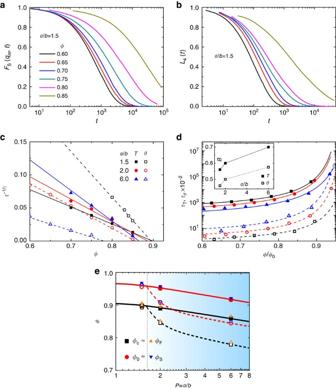Figure 4: The simulation counterpart ofFig. 2. (a)Fs(qm,t) and (b)L4(t) for ellipsoids with aspect ratioP=a/b=1.5. (c) The translational relaxation time τT(solid symbols) and rotational relaxation time τθ(open symbols) fitted with equation (1). (d) τTand τθfitted with equation (2). Symbols are the same as in (c). Inset: the fitted fragility indexB. (e) The measuredϕc,ϕ0,ϕFandϕSfor translational (solid symbols) and rotational (open symbols) motion in simulations all show a single-step glass transition atP≲1.7 and a double-step transition atP≳2.5. Figure 4e shows the crossover from the single-step glass transition to the double-step glass transition at P ≃ 1.7, which is lower than the experimental value 2.5. We attribute this to the following two reasons: (1) an ellipsoid carries a layer of water owing to the stick boundary condition, making its effective size larger and effective P smaller in experiments; (2) surface electric charges on spheres tend to redistribute towards the two ends of the resulting ellipsoids, which reduces the experimental P . Figure 4: The simulation counterpart of Fig. 2 . ( a ) F s ( q m , t ) and ( b ) L 4 ( t ) for ellipsoids with aspect ratio P = a / b =1.5. ( c ) The translational relaxation time τ T (solid symbols) and rotational relaxation time τ θ (open symbols) fitted with equation (1). ( d ) τ T and τ θ fitted with equation (2). Symbols are the same as in ( c ). Inset: the fitted fragility index B . ( e ) The measured ϕ c , ϕ 0 , ϕ F and ϕ S for translational (solid symbols) and rotational (open symbols) motion in simulations all show a single-step glass transition at P ≲ 1.7 and a double-step transition at P ≳ 2.5. Full size image DHs DHs arise from the emergence of domains that are rearranged in a correlated manner and at different rates [1] , [2] . It is characterized by the cooperatively rearranging regions (CRRs), which are closely related to the macroscopic properties of a glass [1] , [36] . CRRs are usually represented by particle clusters with FT motion, which have been well studied in systems of spheres [18] , [36] , [37] , [38] . But much less is known about CRRs that are represented by particle clusters with FR [22] , ST [13] , [15] , [37] and SR [14] motion. Here we directly visualized the spatial distributions of the FT, FR, ST and SR motions of anisotropic particles ( Fig. 5a,b,d,e ). The fastest-moving particles are defined as those with ~8% of the largest displacements during the cage-breaking time τ 2 measured from the peak of the non-Gaussian parameter of displacements Δ x : α 2 ( t )=‹ Δ x 4 › /(3‹ Δ x 2 › 2 ) [18] , [22] , [39] . The measured long-time diffusion coefficient D ( ϕ ) ∝ τ 2 ( ϕ ) −1 holds for all densities and P ’s. Hence τ 2 corresponds to the diffusion time scale [37] . The ~8% corresponds to the non-Gaussian long tails of the displacement distribution. Different percentages of fast and slow particles yield similar results. The slowest-moving particles are defined as those with Δ r 2 (τ T )<MSD( )/4 for translation motion and Δ θ 2 (τ θ )<MSD( )/4 for rotation motion, where t * corresponds to the middle of the mean-square displacement (MSD) plateau. can be regarded as a measurement of cage size [37] , [40] . Fast and slow particles formed the largest clusters at the cage-breaking time τ 2 (ref. 18 ) and the structural relaxation time τ [37] , respectively. Consequently the fastest-moving particles are defined as those with the largest displacements during τ 2 since they dominate diffusion [39] , while the slowest-moving particles are defined as those with the smallest displacements during τ since they dominate the structural relaxation [37] . For the two samples with the highest ϕ ’s, the slow particles are defined at the longest experimental time because their τ are longer than the experimental time. This leads ξ S to be only slightly underestimated at the two highest ϕ ’s because the longest experimental time is on the same order of magnitude as τ. Subsequently, we can identify the FT, FR, ST and SR clusters by using the criterion that two fast (or slow) particles belong to the same cluster if they are neighbours. Here we define two ellipsoids as neighbours when they overlap after expanding by 1.5 times and no other particles intersect at their closest distance [22] . 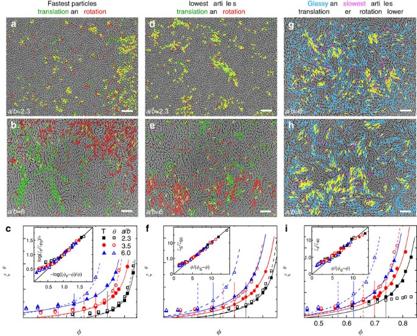Figure 5: Fast, slow and glassy clusters. Spatial distributions of translational (green ~8%) and rotational (red ~8%) fastest (a,b) and slowest (d,e) particles, and of translational (g) and rotational (h) glassy (blue ~30%) and slowest (pink ~10%) particles. Particles that are fast (or slow) in both translational and rotational motion (a,b,d,e) or that are both slow and glassy (g,h) are labelled in yellow. Scale bar, 20 μm. (a,d), (b,e) and (g,h) are taken from the same frame atϕ=0.81,P=2.3;ϕ=0.70,P=6 andϕ=0.74,P=6, respectively. (c) The characteristic size of fast clusters (symbols) fitted with equation (3) (curves). Inset: the data points collapse onto a master curve with unit slope in the logarithmic plot. (f) The characteristic size of slow clusters (symbols) fitted with equation (4) (curves). Inset: the data points collapse onto a master curve with unit slope in the logarithmic plot. (i) The characteristic size of glassy clustersξg(main panel) and the four-point dynamic correlation lengthξ4(inset). Both sets of data are well fitted with equation (4), except foratP=2.3. The vertical lines in (c,f,i) mark the onsets of dynamic heterogeneities, below which the data points deviate from the fitting curves. Figure 5: Fast, slow and glassy clusters. Spatial distributions of translational (green ~8%) and rotational (red ~8%) fastest ( a , b ) and slowest ( d , e ) particles, and of translational ( g ) and rotational ( h ) glassy (blue ~30%) and slowest (pink ~10%) particles. Particles that are fast (or slow) in both translational and rotational motion ( a , b , d , e ) or that are both slow and glassy ( g , h ) are labelled in yellow. Scale bar, 20 μm. ( a , d ), ( b , e ) and ( g , h ) are taken from the same frame at ϕ =0.81, P =2.3; ϕ =0.70, P =6 and ϕ =0.74, P =6, respectively. ( c ) The characteristic size of fast clusters (symbols) fitted with equation (3) (curves). Inset: the data points collapse onto a master curve with unit slope in the logarithmic plot. ( f ) The characteristic size of slow clusters (symbols) fitted with equation (4) (curves). Inset: the data points collapse onto a master curve with unit slope in the logarithmic plot. ( i ) The characteristic size of glassy clusters ξ g (main panel) and the four-point dynamic correlation length ξ 4 (inset). Both sets of data are well fitted with equation (4), except for at P =2.3. The vertical lines in ( c , f , i ) mark the onsets of dynamic heterogeneities, below which the data points deviate from the fitting curves. Full size image The FT, FR, ST and SR clusters exhibit different novel correlations at P ≳ 2.5 and P ≲ 2.5. In Fig. 5a,b , we labelled the fastest translational particles in green and the fastest rotational particles in red. The particles fast in both translational and rotational motion are labelled in yellow. In Fig. 5d,e , ellipsoids are similarly labelled for slowest particles. The FT, FR, ST and SR particles clearly show different positive or negative correlations in Fig. 5a,d ( P =2.3) and in Fig. 5b,e ( P =6.0). For P ≳ 2.5, the four types of clusters are all anticorrelated in space and the anticorrelations become stronger as P increases due to better developed nematic domains ( Fig. 5b,e ). For P ≲ 2.5, by contrast, positive correlations are observed between FT and FR clusters and between ST and SR clusters as can be appreciated from the fact that most of the clusters are now coloured yellow in Fig. 5a,d . 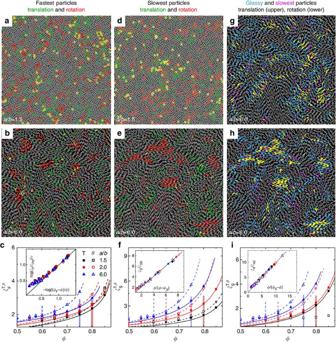Figure 6: The simulation counterpart ofFig. 5. The spatial distributions of translational (green) and rotational (red) fast (a,b) and slow (d,e) particles. (g,h) Glassy particles (blue) and slow particles (pink) in translational (g) and rotational (h) motion. Particles that are fast (or slow) in both translational and rotational motion (a,b,d,e) or that are both slow and glassy (g,h) are labelled in yellow. Ellipsoids are plotted as 0.8 times their real size (that is, 0.64 times their real area) for clarity. (a,d), (b,e) and (g,h) are taken from the same frame atϕ=0.85,P=1.5;ϕ=0.80,P=6 andϕ=0.80,P=6, respectively. (c) The characteristic sizes of fast clusters (symbols) fitted with equation (3) in the main text (curves). (f) The characteristic sizes of slow clusters (symbols) fitted with equation (4) in the main text (curves). (i) The characteristic sizes of glassy clustersξg(main panel) and the four-point dynamic correlation lengthξ4(inset). Both sets of data are well fitted with equation (4), except for the rotational motion atP=1.5. The data points in (c,f,i) collapse onto a master curve in the logarithmic plot in the insets. The solid and dashed vertical lines in (c,f,i) mark the onsets of DHs, below which the data points deviate from the fitting curves. Figure 6 is the simulation counterpart of Fig. 5 . It shows the same results of the spatial distribution and correlations of the FT, FR, ST and SR particles. The slow and fast particles in Fig. 6 cover about 10% of all particles. The percentage of overlap of fast (or slow) transitional and rotational particles (that is, the ratio of yellow to (red+yellow) particles) is about 20% (>10%) at P =1.5 and 5% (<10%) at P =6.0, which indicates positive and negative correlations, respectively. Figure 6: The simulation counterpart of Fig. 5 . The spatial distributions of translational (green) and rotational (red) fast ( a , b ) and slow ( d , e ) particles. ( g , h ) Glassy particles (blue) and slow particles (pink) in translational ( g ) and rotational ( h ) motion. Particles that are fast (or slow) in both translational and rotational motion ( a , b , d , e ) or that are both slow and glassy ( g , h ) are labelled in yellow. Ellipsoids are plotted as 0.8 times their real size (that is, 0.64 times their real area) for clarity. ( a , d ), ( b , e ) and ( g , h ) are taken from the same frame at ϕ =0.85, P =1.5; ϕ =0.80, P =6 and ϕ =0.80, P =6, respectively. ( c ) The characteristic sizes of fast clusters (symbols) fitted with equation (3) in the main text (curves). ( f ) The characteristic sizes of slow clusters (symbols) fitted with equation (4) in the main text (curves). ( i ) The characteristic sizes of glassy clusters ξ g (main panel) and the four-point dynamic correlation length ξ 4 (inset). Both sets of data are well fitted with equation (4), except for the rotational motion at P =1.5. The data points in ( c , f , i ) collapse onto a master curve in the logarithmic plot in the insets. The solid and dashed vertical lines in ( c , f , i ) mark the onsets of DHs, below which the data points deviate from the fitting curves. Full size image The development of DHs can be characterized by the increasing sizes of fast and slow clusters. We found that the characteristic size ξ F of fast clusters is best fitted with [2] , [38] , [39] : which diverges at ϕ F ( Figs 5c and 6c ); while the characteristic size ξ S of slow clusters is best fitted with which diverges at ϕ S ( Figs 5f and 6f ). N F , S are the numbers of particles in a fast cluster and a slow cluster, respectively. Equation (4) is consistent with the scaling argument in ref. 4 . The experimental fitting exponents ν =0.72, 0.59 and 0.448 for and ν =0.75, 0.625 and 0.48 for at P =2.3, 3.5 and 6.0, respectively, and the simulation ν =0.38, 0.345 and 0.29 for and ν =0.43, 0.385 and 0.33 for at P =1.5, 2.0 and 6.0, respectively. These trends indicate that the size of CRRs grows faster in more fragile glassy systems. ξ F ( ϕ ) can be better fitted by a slightly different form, , in a broader range of ϕ , but we fit Figs 5c and 6c with equation (4) since it follows ( T eff − ) − ν in MCT where ~1/ ϕ for colloids. and obtained from the best fits of equations (3 and 4) are almost identical to and , respectively for all P ’s ( Fig. 2e ), in accordance with the fact that free diffusions dominated by fast particles become kinetically arrested at the mode-coupling critical density ϕ c , and structural relaxations dominated by slow particles cease at the ideal glass transition density ϕ 0 . Above ϕ F ≃ ϕ c , the fast particles dispersed randomly because they were all caged separately [18] . Moreover, we observe from the insets of Fig. 5f,i that the characteristic size of slow clusters ξ S reflects the length scale of DHs, which is typically characterized by the dynamic correlation length ξ 4 obtained from the four-point density correlation function [2] , [28] . The insets of Figs 5i and 6i show that ξ 4 ∝ ϕ /( ϕ 0 − ϕ ) [13] is identical to equation (4) since our ϕ S ≃ ϕ 0 . Hence ξ S ( ϕ ) ∝ ξ 4 ( ϕ ) for both translational and rotational motion and for all P ’s. The structure–dynamics relationship First, we probe the static structure by identifying the glassy particles and show that the glassy clusters are highly correlated to the dynamic slow clusters in both translational and rotational degrees of freedom. Glassy particles are defined as local static structures with strong cage effects. We define a particle with N n ≥6 nearest neighbours as translational glassy, and a particle with a local orientational order as rotational glassy, where Δ θ j is the angle difference between the particle and its j th neighbour. In practice, the glassy particles in Figs 5g,h and 6g,h are defined from the structures averaged over τ for better statistics: for translational glassy particles and for rotational glassy particles. Such an average was used in refs 13 , 14 and is reasonable since slow particles are defined over the structural relaxation time τ. Note that N n and S n are still static quantities after the time averaging. Without time averaging, the positive spatial correlations can also be resolved, but with a larger noise. N n and S n in Figs 5i and 6i are defined without time average. Rotational glassy particles have a high local nematic orientational order, but the translational glassy particles do not exhibit apparent positional order (see the three typical configurations with some splay structures in Fig. 7 ). 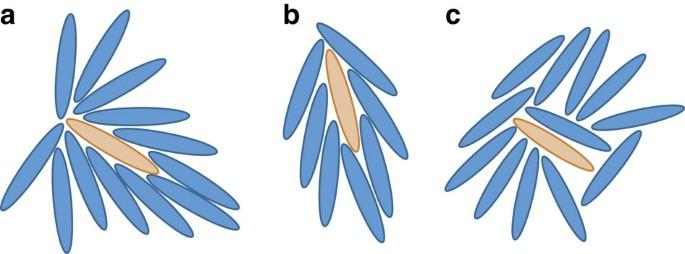Figure 7: Typical configurations with splay structures. a,bandcexhibit some splay structures around a translational glassy particle (in orange) with high number of nearest neighbours. Figure 7: Typical configurations with splay structures. a , b and c exhibit some splay structures around a translational glassy particle (in orange) with high number of nearest neighbours. Full size image N n and S n exhibited broader probability distributions, that is, more structural disorder and stronger frustration, at larger P . This observation confirmed the expectation that the lower dynamic fragility (inset of Fig. 2d ) arises from the stronger structural frustration [5] , [13] . The complex local structures in an ellipsoid system ( Fig. 7 ) make it difficult to identify whether it is geometrical frustration [5] or frustration due to competing order [8] , [13] , [14] . For geometrical frustration, the slow dynamics corresponds to the local stable structure (for example, icosahedral order) that cannot tile the whole space, while the slow dynamics corresponds to the global stable structure (for example, crystalline order) in competing-order frustration. In ellipsoids, however, a local favourable structure is ambiguous. The close packing of three ellipsoids tends to form a splay structure as shown in Fig. 1f , but close packing of more ellipsoids will form different structures ( Fig. 7 ). Hence the observed slow clusters ( Figs 5d,e and 6d,e ) contain various complex structures without a particular crystalline or amorphous order. The fraction of glassy particles increases with packing fraction ϕ up to 30% at our highest ϕ , while the fraction of slow particles remains at around 8%. These particles have strong positive correlation in space ( Figs 5g,h and 6g,h ). When P ≳ 2.5, translational and rotational glassy clusters are spatially anticorrelated: translational glassy particles are mainly found at domain boundaries, while rotational glassy particles are mainly inside one or multiple adjacent nematic domains. The number of particles in a translational (or rotational) glassy cluster is denoted as (or ). The mean glassy-cluster size can be well fitted with ( Figs 5i and 6i ), except for the rotational glassy clusters at P =2.3 ( Figs 5i and 6i ), since this system lacks nematic domains ( Figs 5a,d and 6a,d ) and the glass transition is dictated by translational motion. The dynamic slowing down is expected to be originated from the decrease in the number of accessible configurations [3] , [4] , [8] . Recently, Tanaka et al. [13] measured the local structural entropy arising from the two-body correlation, s 2 , in translational degree of freedom in systems of hard spheres. They showed that crystalline clusters have a lower structural entropy and their sizes have the same power-law divergence as the correlation length of DH when approaching the glass transition [13] . Here we similarly explore whether glassy clusters are related to low structural entropy in systems of ellipsoids. s 2 of an ellipsoid i comprises the translational and rotational entropies, , which can be evaluated as [41] , [42] where k B is the Boltzmann constant, ρ is the number density, g i ( r ) is the radial distribution function of centers of mass relative to particle i , g i ( θ | r ) is the orientational distribution function of the angular difference between the long axis of particle i and its neighbouring particle at center-of-mass distance r [42] . The free-volume entropies from multiple layers of neighbours are included in equations (5 and 6) via the weights of g i ( r ) and g i ( θ | r ). Both the experiments ( Fig. 8a–d ) and the simulations ( Fig. 9a–d ) show that the static low-structural-entropy particles and the glassy particles are strongly correlated in both translational and rotational degrees of freedom. Note that previous studies found no correlations between DHs and the local free volume in the nearest layer [43] , [44] . By contrast, s 2 contains the free-volume effect from several layers of neighbours instead of only the nearest layer, and remarkably reveals the correlations with DHs. 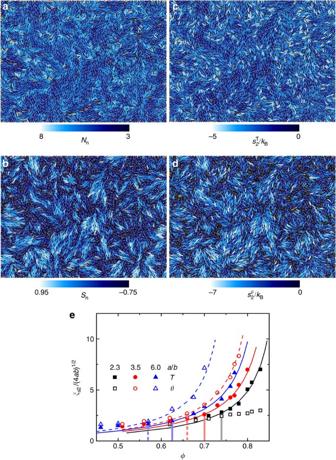Figure 8: Spatial distributions and correlations of local structural entropy. (a–d) The same frame of ellipsoids with aspect ratioP=6 atϕ=0.74. (a) The spatial distributions of (a) the number of nearest neighboursNn, (b) the local nematic orderSn, (c) the translational structural entropyand (d) the orientational structural entropy.aandcexhibit similar distributions, as dobandd. (e) The correlation length offitted withξs2=ξs20·ϕ/(ϕ0−ϕ). Only the rotational motion for ellipsoids withP=2.3 deviates from the fitting curve as inFig. 5i. (a–d) are not time averaged, while (i) is time averaged over the β-relaxation time for lower noises. Figure 8: Spatial distributions and correlations of local structural entropy. ( a – d ) The same frame of ellipsoids with aspect ratio P =6 at ϕ =0.74. ( a ) The spatial distributions of ( a ) the number of nearest neighbours N n , ( b ) the local nematic order S n , ( c ) the translational structural entropy and ( d ) the orientational structural entropy . a and c exhibit similar distributions, as do b and d . ( e ) The correlation length of fitted with ξ s 2 = ξ s 20 · ϕ /( ϕ 0 − ϕ ). Only the rotational motion for ellipsoids with P =2.3 deviates from the fitting curve as in Fig. 5i . ( a – d ) are not time averaged, while ( i ) is time averaged over the β-relaxation time for lower noises. 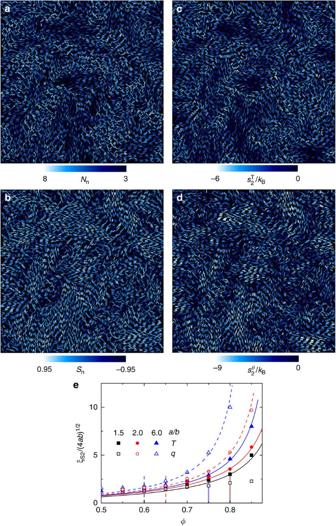Figure 9: The simulation counterpart ofFig. 8. (a–d) The same frame of ellipsoids with aspect ratioP=6 atϕ=0.80. The spatial distributions of (a) the number of nearest neighboursNn, (b) the local nematic orderSn, (c) the translational structural entropyand (d) the orientational structural entropy.aandcexhibit similar distributions, as dobandd. (e) The correlation length offitted withξs2=ξs20·ϕ/(ϕ0−ϕ). Only the rotational motion for ellipsoids withP=1.5 deviates from the fitting curve as inFig. 6i. (a–d) are not time averaged, while (i) is time averaged over the β-relaxation time for lower noises. Full size image Figure 9: The simulation counterpart of Fig. 8 . ( a – d ) The same frame of ellipsoids with aspect ratio P =6 at ϕ =0.80. The spatial distributions of ( a ) the number of nearest neighbours N n , ( b ) the local nematic order S n , ( c ) the translational structural entropy and ( d ) the orientational structural entropy . a and c exhibit similar distributions, as do b and d . ( e ) The correlation length of fitted with ξ s 2 = ξ s 20 · ϕ /( ϕ 0 − ϕ ). Only the rotational motion for ellipsoids with P =1.5 deviates from the fitting curve as in Fig. 6i . ( a – d ) are not time averaged, while ( i ) is time averaged over the β-relaxation time for lower noises. Full size image We measure the spatial correlation of s 2 , , and fit it with the 2D Ornstein–Zernike correlation function [13] , [45] to obtain the correlation length ξ s 2 . ξ s 2 in Figs 8e and 9e are averaged over β-relaxation time τ β .τ β is fitted from the critical-decay law in the β-relaxation, where the nonergodicity parameter and the amplitude h q are constant [27] . Averaging over τ β was also performed when defining static crystalline structures for better statistics in ref. 46 and was shown to be short enough to avoid possible mix up of the static and the dynamic effects. Figure 8e shows that ξ s2 has the same scaling as Fig. 5f,i and the inset of Fig. 5i for all P ’s, hence ξ s2 ( ϕ ) ∝ ξ g ( ϕ ) ∝ ξ S ( ϕ ) ∝ ξ 4 ( ϕ ), with all the proportionality prefactors around 1 for both translational and rotational motion. Consequently the Vogel–Fulcher–Tammann equation τ( ϕ ) ∝ exp[ B? /( ϕ 0 − ϕ )]=exp[ B ξ s2 / ξ s20 ]=exp[ B ξ g / ξ g0 ] indicates that the kinetic slowing down is related to the decrease in the local structural entropy and the increase in the size of the glassy clusters. Our experiments and simulations show that the correlation lengths of the local structural entropy, glassy clusters, slow clusters and the four-point dynamic correlation length are all of the same order, ξ s2 ( ϕ ) ∝ ξ g ( ϕ ) ∝ ξ S ( ϕ ) ∝ ξ 4 ( ϕ ), with the same power-law divergence at ϕ 0 in both translational and orientational degrees of freedom. This set of static-dynamic relations and strong spatial correlations of the corresponding clusters in Figs 5 , 6 , 8 and 9 suggest that the static glassy clusters ( ξ g ( ϕ )) corresponding to the static low structural entropy ( ξ s2 ( ϕ )) should be the cause of the slow dynamics ( ξ S ( ϕ )) and the increasing DHs ( ξ 4 ( ϕ )) rather than a series of coincidences. This may suggest that the glass transition has a thermodynamic origin rather than a purely dynamic origin. The power-law divergence of the static correlation length with exponent −1 suggests that the glass transition is probably a 2D Ising-type critical phenomenon [8] , [13] , [15] , [47] , [48] rather than a random first-order transition scenario [2] , in which the dynamical correlation length grows much faster than the static correlation lengths. Moreover, the random first-order transition theory concerns positional order and not orientational order [8] , while the scaling of our orientational S n is more consistent with critical behaviour. In addition, we observed for the first time the crossover from a single-step to a double-step glass transition in a system of anisotropic particles. The glass transitions for translational and rotational motion occur at the same density when the aspect ratio P <2.5, but at different densities when P >2.5 where local nematic domains start to develop. The translational and rotational CRRs exhibit different correlations at P <2.5 and P >2.5. Moreover, ellipsoids with a larger aspect ratio lead to stronger frustration and a reduced fragility. All the experimental results are confirmed by kMC simulations of hard ellipses in 2D. These results show that the shape anisotropy of the particles has important effects on the phase behaviour and dynamics of the resulting glasses. A monolayer of uniformly sized ellipsoids is arguably the simplest glass. Note that uniformly sized hard disks can only form crystals in 2D. This simple yet versatile glass-forming system with measurable translational and rotational dynamics at the single-particle level serves as a valuable test bed on which new insights into glass transitions in molecular systems can be derived. The observed glassy structure and the corresponding CRRs at different aspect ratios cast new light on some novel phenomena such as photomechanical effects, shape memory and excess scattering in molecular, polymeric and liquid-crystal glassy systems [49] , [50] , [51] , [52] , where local orientationally ordered domains play an important role. Our results pave the way towards a deeper understanding of the glass transition in molecular systems. We expect to find similar results in molecular glasses composed of non-spherical particles. Ellipsoids fabrication We fabricated ellipsoids by stretching non-cross-linked PMMA spheres (microparticles GmbH, Berlin) in air using a previously described method [26] , [53] that is upgraded from stretching spheres in hot oil [54] . Briefly, PMMA spheres (0.5% by weight) were added to an aqueous solution of polyvinyl alcohol (PVA) (12% by weight) in a Petri dish. After water evaporation, the solid PVA film was taken out of the Petri dish and stretched at 130 °C, which is above the glass transition temperatures of PVA ( T g =85 °C) and PMMA ( T g =105 °C). The PMMA spheres embedded in the PVA film were thus stretched into ellipsoids. After cooling to room temperature, the PVA was dissolved and washed away with deionized water. The cleaned ellipsoid suspension was stabilized with 7 mM sodium dodecyl sulphate. The Debye layer was thin and the surface charges had minor effects. From the 2D Gaussian fitting of the images of >200 isolated ellipsoids in a dilute monolayer, we obtained the semi-major axis a and semi-minor axis b as fitting parameters. We made four batches of ellipsoids with aspect ratios P = a / b =1.76 μm/0.77 μm=2.3, P =2.33 μm/0.67 μm=3.5, P =3.33 μm/0.56 μm=6.0 and P =4.39 μm/0.49 μm=9.0. The polydispersity of the aspect ratio was 5–6% for all P ’s. Sample cells A monolayer of ellipsoids was dispersed in a thin sample cell composed of two parallel glass plates. Glass surfaces of the sample cell were rigorously cleaned in a 1:4 mixture of hydrogen peroxide and sulphuric acid by sonication. Then the glass was thoroughly rinsed in deionized water. To prepare a 2D sample, a 0.5-μl droplet of the suspension was placed on a glass slide and then a coverslip was placed over it. The droplet spread into a thin film by capillary forces. The ellipsoids did not stick to the surfaces. The sample cell was sealed with epoxy glue. The area fraction was set by holding the cells up vertically for several hours to 1 day so that particles slowly drifted downwards under gravity. When the desired area fraction was reached in the ~mm 2 chosen area, the cells were laid flat on the microscope stage for 2–3 h for equilibration. Two-hour and 24-h equilibration resulted in almost the same area fraction, thus the systems were in metastable equilibrium. We monitored the central ~(0.3 mm) 2 area for 3–6 h at each density. The area fraction remained constant during the whole observation period. For each aspect ratio, we measured 3–5 densities in one sample cell and a total of 12 different densities in three cells. The wall separation was a constant for different densities in one cell because we chose a fixed observation area. The wall separations in different cells were almost the same since dilute ellipsoids have the same diffusion coefficients. Under the strong confinement, the heavy ellipsoids always stayed in the focal plane and the fluctuation in the z direction was very weak. The tips of ellipsoids occasionally overlapped, which shifts the glass transition points to <2% area fraction higher. For brevity, we use the term 2D instead of quasi-2D in the main text. The center-of-mass positions and the orientations of individual ellipsoids were tracked using our image-processing algorithm [26] . The angular resolution was 1°, and the spatial resolutions were 0.12 and 0.04 μm along the long and short axes, respectively. We projected each step of displacement measured in lab frame to the body frame, then connected all steps into a trajectory along the long and short axes [53] so that transverse motion and longitudinal motion can be separately tracked. ξ 4 ( t ). We calculated the dynamic correlation length ξ 4 ( t ) from the four-point density correlation function as follows. The four-point correlation function of the overlapping particles is defined as , where ρ is the number density. The overlapping function w | r 1 − r 2 | is unity if | r 1 − r 2 |≤0.2 a for translation and | θ 1 − θ 2 |≤0.1 π for rotation and zero otherwise. We calculated the four-point structure factor of overlapping particles as the Fourier transform of g 4 ( r , t ): S 4 ( q , t )=∫ g 4 ( r , t )exp[− i q · r ] d r . To extract ξ 4 at t =τ, we fitted S 4 with S 4 ( q ,τ)= S 0 /[1+( ξ 4 q ) 2 ] [28] . The fitted ξ 4 ’s are shown in the insets of Figs 5i and 6i . Simulation We performed kMC simulations to mimic the Brownian motion of 5,000 ellipses. In each kMC step, we randomly generated three types of trial moves: translational displacement along the long axis δ a , translational displacement along the short axis δ b and rotational displacement δ θ . δ a follows the uniform random distribution in [−Δ a ,Δ a ]. δ b and δ θ were similarly generated. The maximum displacements Δ satisfy where P ( δ a ), P ( δ b ) and P ( δ θ ) are the acceptance ratios for the displacements δ a , δ b and δ θ , respectively. We employed the algorithm in ref. 55 to check the extent of overlap of two hard ellipsoids and obtained the acceptance ratios from the simulation. The ratios between the short-time diffusion coefficients D a , D b and D θ were adopted from the experiments. We also performed simulations with different ratios and further confirmed that the short-time dynamics of individual particles does not affect the dynamics of the system close to the glass transition points. After N MC MC steps, we have and D =( D a + D b )/2, thus the duration of each MC step Δ t in the unit of the Brownian time τ B can be derived as where τ B is the time taken for an ellipsoid to diffuse a distance b in an infinitely dilute suspension. How to cite this article: Zheng, Z. et al. Structural signatures of dynamic heterogeneities in monolayers of colloidal ellipsoids. Nat. Commun. 5:3829 doi: 10.1038/ncomms4829 (2014).